Fermi-surface reconstruction by stripe order in cuprate superconductors The origin of pairing in a superconductor resides in the underlying normal state. In the cuprate high-temperature superconductor YBa 2 Cu 3 O y (YBCO), application of a magnetic field to suppress superconductivity reveals a ground state that appears to break the translational symmetry of the lattice, pointing to some density-wave order. Here we use a comparative study of thermoelectric transport in the cuprates YBCO and La 1.8−x Eu 0.2 Sr x CuO 4 (Eu-LSCO) to show that the two materials exhibit the same process of Fermi-surface reconstruction as a function of temperature and doping. The fact that in Eu-LSCO this reconstruction coexists with spin and charge modulations that break translational symmetry shows that stripe order is the generic non-superconducting ground state of hole-doped cuprates. In the underdoped region of the phase diagram, quantum oscillations have revealed a small Fermi surface pocket in the cuprate superconductor YBCO (ref. 1 ), in contrast to the large Fermi surface observed on the overdoped side. This implies that there is a quantum critical point (QCP) near optimal doping where the Fermi surface of the non-superconducting ground state is reconstructed. Understanding this QCP is essential, and if it corresponds to the onset of some density-wave order that breaks the translational symmetry of the CuO 2 planes, then the fluctuations of that order may well cause both the linear temperature dependence of the resistivity in the 'strange-metal phase' and the pairing [2] . Such a density-wave scenario applies to organic superconductors [3] , for example, and possibly also to iron-pnictide and heavy-fermion superconductors [4] . In cuprates, the nature and origin of the small Fermi pocket are the subject of much debate [5] . An electron-like rather than hole-like pocket would strongly favour a density-wave scenario whereby the Fermi surface undergoes a reconstruction driven by the new periodicity [6] , [7] , as in the case of antiferromagnetism [8] , d -density-wave order [9] , or stripe order [10] . Here we report quantum oscillations in the Seebeck and Nernst coefficients of YBCO and show, from the magnitude and sign of the Seebeck coefficient, that they come from an electron pocket. Using measurements of the Seebeck coefficient as a function of hole doping p , we show that the evolution of the Fermi surface in YBCO is the same as in Eu-LSCO, a cuprate where stripe order—a modulation of spin and charge densities [11] , [12] —is well established [13] , [14] , [15] , [16] . The electron pocket is most prominent where stripe order is strongest, at p =1/8. This shows that Fermi-surface reconstruction is a generic mechanism of underdoped cuprates, intimately related to stripe order. Quantum oscillations Quantum oscillations in YBCO at a hole doping p ≈0.1 have a dominant frequency F ≈530 T (refs 1 , 17 , 18 ), giving a closed Fermi surface area 30 times smaller than that found in overdoped Tl 2 Ba 2 CuO 6+y at p ≈0.3 (ref. 19 ). A key question is the sign of the associated carriers. The large negative Hall coefficient R H observed in the same YBCO samples at low temperature is evidence of electron-like carriers [20] , [21] . However, because a negative Hall resistance can, in principle, come from moving vortices or negative curvature in a hole-like Fermi surface, it is important to confirm the sign of carriers using evidence insensitive to these effects. This can be done by measuring the Seebeck coefficient (or thermopower) S , a standard measure of carrier sign. 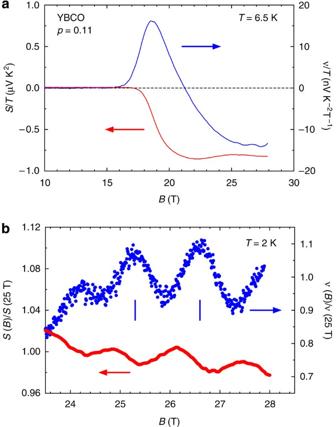Figure 1: Quantum oscillations in the thermoelectric response of YBCO. (a) Seebeck (S; red curve, left axis) and Nernst (ν; blue curve, right axis) coefficients of YBCO measured in a single crystal with a dopingp=0.11 at a temperatureT=6.5 K, plotted asS/Tand ν/Tvs magnetic fieldB. (b) Zoom on the high-field range of the same coefficients, measured atT=2 K, normalized to their respective values atB=25 T. Quantum oscillations are clearly seen in both coefficients. The short vertical lines show the spacing of two successive oscillations of frequencyF=520 T (in 1/B). In Figure 1a , we show S and the Nernst coefficient ν of YBCO at p =0.11, measured at low temperature as a function of magnetic field B up to 28 T. The fact that ν is flat at high field shows that vortex contributions have become negligible above 25 T, and the normal state has for all practical purposes been reached. The fact that S is negative in that high-field normal state confirms that the dominant carriers are electron-like. Figure 1: Quantum oscillations in the thermoelectric response of YBCO. ( a ) Seebeck ( S ; red curve, left axis) and Nernst (ν; blue curve, right axis) coefficients of YBCO measured in a single crystal with a doping p =0.11 at a temperature T =6.5 K, plotted as S / T and ν/ T vs magnetic field B . ( b ) Zoom on the high-field range of the same coefficients, measured at T =2 K, normalized to their respective values at B =25 T. Quantum oscillations are clearly seen in both coefficients. The short vertical lines show the spacing of two successive oscillations of frequency F =520 T (in 1/ B ). Full size image A zoom on the data at 2 K ( Fig. 1b ) reveals quantum oscillations in both S and ν , proving the presence of a small closed pocket in the Fermi surface of YBCO in fields as low as 24 T. The frequency of the oscillations (in 1/ B ) is F ≈520 T, in agreement with quantum oscillations in the resistance [1] and magnetization [17] , [18] of similar YBCO crystals. Given a cyclotron mass m *=1.76±0.07 m 0 (ref. 17 ), we obtain the Fermi temperature T F =( eħ / k B ) ( F / m *)=410±20 K, where m 0 and e are the electron mass and charge, respectively, and k B is the Boltzmann constant. From T F , we estimate the magnitude of the Seebeck and Nernst coefficients expected for this Fermi pocket at T →0, using standard expressions known to agree well with experiment in several correlated electron systems. These yield (ref. 22 ): where the negative sign is for electron-like carriers. The upper and lower bounds on the uncertainty correspond to assuming an energy-independent relaxation time ( ζ =0) or mean-free path (ζ=−1/2), respectively [22] . The measured value at low temperature is S / T =−0.8±0.1 μV K −2 ( Fig. 1a ). The magnitude of the quasiparticle Nernst coefficient at T →0, ν / T =−13±3 nV K −2 T−1 ( Fig. 1a ), is also the expected value [23] given the mobility μ=0.02±0.006 T −1 obtained from quantum oscillations [17] . This excellent quantitative agreement shows that, in YBCO at p =0.11, the quantum oscillations come from a small electron-like Fermi pocket of high mobility. 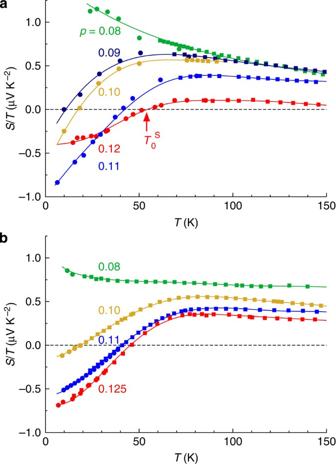Figure 2: Seebeck coefficient of YBCO and Eu-LSCO. (a) Normal-state Seebeck coefficient of YBCO, plotted asS/TvsT, measured in a fieldB=0 (squares) andB=28 T (circles), at five values of the hole dopingpas indicated (data atp=0.12 from ref.37).T0Sis the temperature whereSchanges sign. (b) Corresponding data for Eu-LSCO, measured in a fieldB=0 (squares) andB=10 T (circles), at four dopings as indicated (data atp=0.125 from ref.37). Our Eu-LSCO data agrees well with previous data38,39. All lines are a guide to the eye. Seebeck coefficient In Figure 2a, b , the normal-state Seebeck coefficient of YBCO and Eu-LSCO, respectively, is plotted as a function of temperature for different dopings. We first discuss the YBCO data. At all dopings, S / T is positive at high temperature. For p =0.09, 0.10, 0.11 and 0.12, S / T starts to drop monotonically below ~80 K, to become negative in the T =0 limit, changing sign at a temperature T 0 S . We infer that an electron pocket is present in the Fermi surface at all four dopings. By contrast, at p =0.08, S / T shows no downturn down to the lowest temperature. The same evolution was reported recently in the Hall coefficient, with R H ( T ) crossing to negative values at a sign-change temperature T 0 H when p >0.08 and remaining positive at p =0.08 (ref. 21 ). The sudden qualitative change in R H ( T ) across p =0.08, now reproduced in S ( T ), is attributed to a change in Fermi surface topology whereby the electron pocket disappears below p =0.08 (ref. 21 ). Figure 2: Seebeck coefficient of YBCO and Eu-LSCO. ( a ) Normal-state Seebeck coefficient of YBCO, plotted as S / T vs T , measured in a field B =0 (squares) and B =28 T (circles), at five values of the hole doping p as indicated (data at p =0.12 from ref. 37 ). T 0 S is the temperature where S changes sign. ( b ) Corresponding data for Eu-LSCO, measured in a field B =0 (squares) and B =10 T (circles), at four dopings as indicated (data at p =0.125 from ref. 37 ). Our Eu-LSCO data agrees well with previous data [38] , [39] . All lines are a guide to the eye. 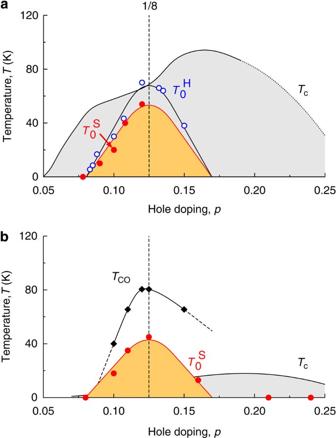Figure 3: Phase diagram of YBCO and Eu-LSCO. (a) Temperature-doping phase diagram of YBCO showing the zero-field superconducting phase belowTc(grey region) and the region where the normal-state Seebeck coefficient is negative (S<0; yellow dome), delineated byT0S(full red circles). Also shown is the line below which the normal-state Hall coefficient is negative (RH<0), calledT0H(open blue circles; ref.21). (b) Phase diagram of Eu-LSCO showingTc(grey region),T0S(full red circles) andTCO, the onset of charge-stripe order detected by X-ray diffraction (full black diamonds; ref.16). Lines throughT0S,T0HandTCOare a guide to the eye. The black vertical dashed line marks the dopingp=1/8. Full size image A convenient way to picture the doping evolution of the Fermi surface is to plot T 0 S on a phase diagram, as shown in Figure 3a for YBCO, and Figure 3b for Eu-LSCO. For YBCO, T 0 S and T 0 H are seen to track each other closely, growing monotonically and in parallel from zero at p =0.08 to their maximal value at p =0.12. Hall measurements up to 60 T reveal that T 0 H comes down at higher doping, so that T 0 H forms a dome starting at p =0.08, peaking at p =1/8, and ending at p ≈0.17 (ref. 21 ). This dome is the region of the phase diagram where the electron pocket dominates the transport properties. Figure 3: Phase diagram of YBCO and Eu-LSCO. ( a ) Temperature-doping phase diagram of YBCO showing the zero-field superconducting phase below T c (grey region) and the region where the normal-state Seebeck coefficient is negative ( S <0; yellow dome), delineated by T 0 S (full red circles). Also shown is the line below which the normal-state Hall coefficient is negative ( R H <0), called T 0 H (open blue circles; ref. 21 ). ( b ) Phase diagram of Eu-LSCO showing T c (grey region), T 0 S (full red circles) and T CO , the onset of charge-stripe order detected by X-ray diffraction (full black diamonds; ref. 16 ). Lines through T 0 S , T 0 H and T CO are a guide to the eye. The black vertical dashed line marks the doping p =1/8. Full size image Two questions arise: is this Fermi-surface evolution unique to YBCO? what causes the Fermi surface to reconstruct below ~80 K? We address these by turning to Eu-LSCO, a cuprate superconductor with a different crystal structure: tetragonal rather than orthorhombic, with single rather than double CuO 2 layers, without CuO chains, in which doping is done by substituting Sr rather than adding oxygen. 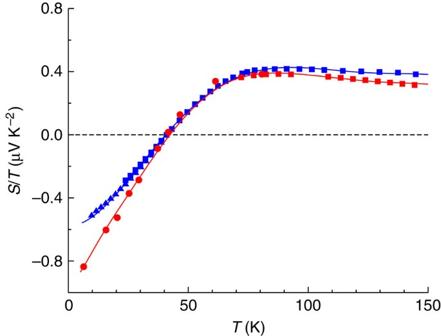Figure 4: Comparing Seebeck data in YBCO and Eu-LSCO. Direct comparison of the Seebeck coefficients of YBCO (red symbols) and Eu-LSCO (blue symbols) at the same doping,p=0.11. The applied magnetic fieldB=0 (squares), 10 T (triangles) or 28 T (circles). The very similar downturn in the normal-state data points to a very similar Fermi-surface reconstruction. In Figure 4 , we compare the normal-state Seebeck coefficient of Eu-LSCO to that of YBCO at the same doping, p =0.11. The two curves are essentially identical: S / T has the same positive value at high temperature; it starts to drop at the same onset temperature near 80 K; it crosses zero at the same temperature T 0 S =40 K; and it reaches a large negative value at T →0 in both cases. (Since S is an intensive quantity, its magnitude is independent of the number of CuO 2 planes per unit cell.) Figure 4: Comparing Seebeck data in YBCO and Eu-LSCO. Direct comparison of the Seebeck coefficients of YBCO (red symbols) and Eu-LSCO (blue symbols) at the same doping, p =0.11. The applied magnetic field B =0 (squares), 10 T (triangles) or 28 T (circles). The very similar downturn in the normal-state data points to a very similar Fermi-surface reconstruction. Full size image Our main finding is that the doping evolution of S / T in Eu-LSCO is fundamentally identical to that of YBCO: at p =0.10, 0.11 and 0.12 it drops to become negative, whereas, at p =0.08, it remains positive down to low temperature ( Fig. 2b ). 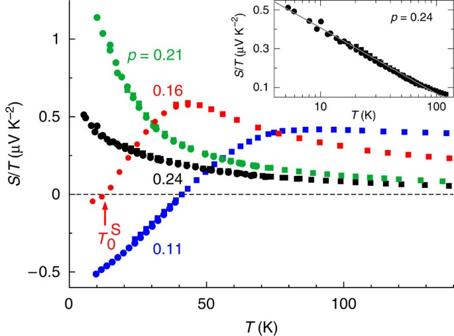Figure 5: Seebeck coefficient of Eu-LSCO at high doping. Normal-state Seebeck coefficientSof Eu-LSCO plotted asS/TvsTfor values of the hole dopingpas indicated, measured in a magnetic fieldB=0 (squares) andB=10 T (circles). Forp=0.16, application of a 10 T field confirms thatSbecomes negative at low temperature, giving a sign-change temperatureT0S≈12 K. Forp=0.21 andp=0.24,S/Tgrows monotonically with decreasing temperature down to the lowest temperature, remaining positive asT→0, so thatT0S=0. Inset:S/Tvs logTforp=0.24. The straight line is a good fit to the data from the lowest temperature (5 K) to ~70 K. This log(1/T) dependence is a signature of a QCP, also observed in La1.6−xNd0.4SrxCuO4atp=0.24 (ref.32). As shown in Figure 5 for Eu-LSCO, a drop to a negative S/T is also observed at p =0.16, whereas, for p =0.21 and 0.24, no drop is seen and S / T is positive at all temperatures. In Figure 3 , a plot of T 0 S versus p captures the striking similarity between Eu-LSCO and YBCO. We conclude that the Fermi surface of these two cuprates undergoes a very similar reconstruction as a function of temperature and doping, pointing to a universal phenomenon amongst hole-doped cuprates. This immediately implies that quantum oscillations and the downturns in S / T and R H come from a Fermi pocket associated with the CuO 2 planes (and not the CuO chains of YBCO, for example). Figure 5: Seebeck coefficient of Eu-LSCO at high doping. Normal-state Seebeck coefficient S of Eu-LSCO plotted as S / T vs T for values of the hole doping p as indicated, measured in a magnetic field B =0 (squares) and B =10 T (circles). For p =0.16, application of a 10 T field confirms that S becomes negative at low temperature, giving a sign-change temperature T 0 S ≈12 K. For p =0.21 and p =0.24, S / T grows monotonically with decreasing temperature down to the lowest temperature, remaining positive as T →0, so that T 0 S =0. Inset: S / T vs log T for p =0.24. The straight line is a good fit to the data from the lowest temperature (5 K) to ~70 K. This log(1/ T ) dependence is a signature of a QCP, also observed in La 1.6−x Nd 0.4 Sr x CuO 4 at p =0.24 (ref. 32 ). Full size image Upon cooling below ~100 K, Eu-LSCO undergoes an ordering process called 'stripe order' [11] , [12] , also observed in the closely related material La 1.6−x Nd 0.4 Sr x CuO 4 (Nd-LSCO), which involves both charge [16] , [24] and spin modulations [13] , [14] , [25] , [26] . These are in general incommensurate with the lattice, with a period of ~4 a and 8 a at p ≈1/8, respectively, where a is the in-plane lattice constant. The charge-ordering temperature T CO in Eu-LSCO is displayed in Figure 3b . At T →0, both modulations are present throughout the doping range 0.10 ≤ p ≤0.15 (refs 13 , 14 , 16 ), and by extrapolation from p ≈0.08 to beyond p ≈0.2. Because they break the translational symmetry of the lattice, these stripe modulations will inevitably cause a reconstruction of the Fermi surface. Calculations show that the reconstructed Fermi surface will in general contain electron pockets [10] . We have now shown that throughout the doping range 0.10≤ p ≤0.16, the Fermi surface of Eu-LSCO does indeed contain an electron pocket. We conclude that stripe order is the mechanism responsible for Fermi-surface reconstruction in Eu-LSCO. By close analogy, we infer that the same mechanism acts in YBCO. By extension, Fermi-surface reconstruction by stripe order is likely to be a generic property of hole-doped cuprates in the approximate range 0.08< p <0.2, and possibly beyond. Apart from the presence of a small closed electron pocket, little is known with certainty about the reconstructed Fermi surface of YBCO or Eu-LSCO. In particular, the k -space location of the electron pocket and the existence of other Fermi-surface sheets are open questions. Studies of the electronic structure by angle-resolved photoemission spectroscopy in Eu-LSCO (ref. 27 ) and Nd-LSCO (ref. 28 ) at p ≈1/8, performed between T c and T CO , revealed evidence of a Fermi-surface reconstruction. However it is unclear whether these effects are due to stripe order or to structural distortions, and no direct evidence for an electron pocket was found. The excellent agreement between the measured value of S / T at T →0 and that calculated assuming the Fermi surface consists of only the electron pocket implies that other Fermi-surface sheets, as yet unobserved, must have a much lower conductivity. In particular, a hole-like sheet would make the Seebeck and Hall coefficients less negative. From the frequency of quantum oscillations in YBCO at p ≈0.1, the Hall coefficient of the electron pocket alone should be R e =−1/ ne =−15 mm 3 C −1 , since n = F /Φ 0 =0.038 carriers per planar Cu atom (ref. 20 ), assuming an isotropic pocket. The measured value of the Hall coefficient is R H =−35 mm 3 C −1 (ref. 20 ). The fact that | R H |>| R e | suggests that the electron pocket is not isotropic, and it leaves little room for a significant hole-like contribution. The contribution of the electron pocket to the normal-state electronic specific heat C e at T →0 is [21] C e pocket / T =( π 2 /2) k B ( n / T F )=5.1±0.2 mJ mol −1 K −2 , where n is the carrier density per unit cell (assuming one electron pocket for each of the two CuO 2 planes in the unit cell). Recent high-field measurements on a YBCO crystal with p ≈0.11 yield C e / T =4−5 mJ mol −1 K −2 above 25 T (ref. 29 ), in agreement with expectation if there are no other sheets in the Fermi surface, or if such sheets have a very low mass m *. Stripe order is known to be most robust at p =1/8, as indicated for example by the fact that the onset temperature T CO is highest at that doping (see Fig. 3b ). Hence, the fact that T 0 S in Eu-LSCO and T 0 H in YBCO peak at p =1/8 is further evidence that Fermi-surface reconstruction and stripe order are linked, in both materials. To our knowledge, diffraction studies in YBCO have not yet been carried out in magnetic fields large enough to suppress superconductivity and directly confirm whether or not the non-superconducting ground state in the doping range 0.09–0.15 does indeed have modulations of spin and/or charge. It is conceivable that the stripe-like spin order observed in YBCO at low temperature up to p ≈0.07 in zero field could persist up to higher p when superconductivity is suppressed by a large enough magnetic field [30] . We stress that stripe order extends well above p =1/8, into the highly overdoped region of the phase diagram. The QCP where the stripe-ordered phase at T =0 ends on the high-doping side is approximately at p ≈0.25 (refs 16 , 25 ). Transport measurements [31] , [32] in Nd-LSCO show clearly that Fermi-surface reconstruction still occurs at p =0.20, but no longer does at p =0.24 (the same is true in Eu-LSCO). The precise location of the QCP is p *=0.235±0.005 (ref. 33 ). The presence of such a QCP has a profound impact on the electronic properties, producing, for example, a linear temperature dependence of the resistivity as T →0 (ref. 31 ), the defining signature of the so-called 'strange-metal phase' of cuprates. Significantly, the strength of the anomalous linear- T scattering in hole-doped cuprates was shown to be directly proportional to T c , the strength of superconductivity [2] , [34] , as found in organic superconductors [3] . YBCO samples YBa 2 Cu 3 O y samples are fully detwinned crystals grown at the University of British Columbia in non-reactive BaZrO 3 crucibles from high-purity starting materials (see ref. 35 ). The hole concentration (doping) p in each sample is tuned by adjusting the oxygen content y . The samples are uncut, unpolished thin platelets, whose transport properties are measured via gold evaporated contacts (of resistance <1 Ω ), in a six-contact geometry. The doping p was determined from a relationship between the superconducting temperature T c and the c -axis lattice constant [36] . The value of T c , defined as the point of zero resistance, is: T c =44.5, 55, 57.3, 61.3 and 66 K for samples with y =6.45, 6.49, 6.51, 6.54 and 6.67, giving p =0.08, 0.09, 0.10, 0.11 and 0.12, respectively. Eu-LSCO samples Single crystals of La 1.8−x Eu 0. 2 Sr x CuO 4 were grown at the University of Tokyo using a travelling float zone technique. The doping p is taken to be equal to the Sr content x , to within±0.005. Electrical contacts (of resistance <0.1 Ω at room temperature) were made using silver epoxy diffused into the surface. The value of T c , defined as the point of zero resistance, is: T c =3, 5, 4, 7, 13, 14 and 9 K for samples with x =0.08, 0.10, 0.11, 0.125, 0.16, 0.21 and 0.24, respectively. Measurement of the thermoelectric coefficients The thermoelectric transport coefficients were measured by applying a steady heat current through the sample (along a direction which we define as the x -axis). In YBCO, the current was along the a -axis of the orthorhombic crystal structure to avoid any contribution from the CuO chains; in Eu-LSCO, the current flowed within the CuO 2 planes. The generated thermal gradient was measured using two uncalibrated Cernox chip thermometers (Lakeshore), referenced to a third, calibrated Cernox. The longitudinal and transverse electric fields were measured using nanovolt preamplifiers and nanovoltmeters. All measurements were performed with the temperature of the experiment stabilized within±10 mK and the magnetic field B swept at a constant rate of 0.4–0.9 T min −1 between positive and negative maximal values, with the heat on. The field was applied normal to the CuO 2 planes ( B || z || c ). As the Seebeck coefficient S is symmetric with respect to the magnetic field, it is obtained by taking the mean value between positive and negative fields: where Δ V x is the difference in the voltage along x measured with and without thermal gradient. This procedure removes any transverse contribution that could appear because of slightly misaligned contacts. The longitudinal voltages and the thermal gradient being measured on the same pair of contacts, no geometric factor is involved. The Nernst coefficient N is antisymmetric with respect to the magnetic field, therefore it is obtained by the difference: where L and w are the length and width of the sample, respectively, along x and y , and V y is the voltage along y measured with the heat current on. This antisymmetrization procedure removes any longitudinal thermoelectric contribution from the sample and a constant background from the measurement circuit. The uncertainty on N comes from the uncertainty in determining the sample dimensions, giving typically an error bar of ±10%. Measurements were performed at the University of Sherbrooke up to 10 or 15 T and at the LNCMI in Grenoble up to 28 T. How to cite this article : Laliberté, F. et al . Fermi-surface reconstruction by stripe order in cuprate superconductors. Nat. Commun. 2:432 doi: 10.1038/ncomms1440 (2011).